Isoniazid resistance without a loss of fitness inMycobacterium tuberculosis The emergence of multi- and extensively drug-resistant tuberculosis (MDR-TB and XDR-TB, respectively) has intensified the critical public health implications of this global disease. The fitness of Mycobacterium tuberculosis ( M.tb. ) strains exhibiting MDR and XDR phenotypes is of fundamental importance in predicting whether the MDR-/XDR-TB epidemic will be sustained across the human population. Here we describe a potential mechanism of M.tb. resistance to the TB drug isoniazid (INH) conferred by loss of a sigma factor, SigI. We demonstrate that the gain of INH resistance in the M.tb. Δ sigI mutant might not diminish the organism's fitness for causing disease. These findings have significant implications when considering the ability of drug-resistant M.tb. strains to initiate untreatable TB epidemics, as it is possible that loss or alteration of SigI function could have a role in the generation of MDR and XDR M.tb. strains of suitable fitness to spread in a community setting. Mycobacterium tuberculosis ( M.tb. ) is an ancient pathogen that has coevolved with humans for tens of thousands of years [1] , and the discovery of antibiotics effective against this organism was a monumental breakthrough in the treatment of tuberculosis (TB) patients. However, as has been the case for many other pathogenic microorganisms, drug-resistant strains of M.tb. have arisen through natural selection within humans receiving antimicrobials. While drug resistance-conferring mutations provide the microbe with a selective advantage in the presence of the drug, these genetic alterations may be associated with a loss of fitness in the drug-free environment, through less-efficient binding of a natural substrate, wasted metabolic energy producing resistance proteins or the sacrifice of a pathway involved in the drug's action [2] . Despite this, multi- and extensively drug-resistant (MDR and XDR, respectively) M.tb. strains have spread beyond populations in which they were selected by inappropriate antimicrobial therapy and into treatment-naive patients, where the strains have shown considerable pathogenicity even among non-immunocompromised hosts, indicating that many drug-resistant M.tb. strains are of sufficient fitness to spread person-to-person [3] , [4] , [5] . Isoniazid (INH) is a bactericidal first-line TB drug with an extremely high potency for members of the M.tb. complex, but not other non-tuberculous mycobacteria [6] . Upon entering tubercle bacilli, INH is activated to form an isonicotinyl-free radical by the bacterium's own peroxidase/catalase enzyme encoded by katG [7] . The INH-free radical reacts with NAD to form an INH–NAD adduct that is a highly potent inhibitor of the essential enzyme InhA, an enoyl-ACP reductase required for mycolic acid biosynthesis [8] , [9] , [10] . Surveys of clinical isolates that demonstrate INH resistance reveal that ∼ 50% have alterations in katG (including complete deletion of the gene), and an additional 25% contain compensatory promoter mutations that upregulate the expression of the inhA gene [11] . Mutations in a small number of other genes encoding activators or regulators of NADH, such as mshA or ndh , have also been described and may account for some clinically observed INH resistance [12] . Thus, about 25% of INH-resistant M.tb. isolates are resistant through undetermined mechanisms. In this study, we describe a novel mechanism of INH resistance in M.tb. We identify a regulatory gene, sigI , that when deleted confers INH resistance by reducing the transcription levels of katG . We further show that M.tb. lacking SigI is not attenuated, but rather hypervirulent, compared with wild-type M.tb. in a mouse model of TB, demonstrating that this SigI-related mechanism of INH resistance is not associated with a loss of fitness in M.tb. Identification of the SigI regulon The M.tb. genome encodes 13 sigma factors, including one principal sigma factor ( sigA ), two principal-like sigma factors ( sigB and sigF ) and ten extracytoplasmic function sigma factors ( sigC – sigM ) [13] . Previous reports on 12 of these sigma factors ( sigA – sigH and sigJ – sigM ) have revealed the basic features of their regulons and how they are utilized by M.tb. to adjust to various environmental conditions, including macrophage and mouse infection models, with most sigma factors involved in the regulation of virulence programmes [13] . Therefore, we investigated the role of the relatively uncharacterized sigma factor SigI in the regulation of M.tb. gene expression and virulence phenotypes. Using quantitative real-time reverse transcription PCR (qRT–PCR), sigI gene expression was examined under various growth phases and stress conditions. sigI transcript levels were increased during stationary phase ( Fig. 1a ) as well as during heat shock ( Fig. 1b ). However, little variation in sigI expression was observed in response to other stress conditions. 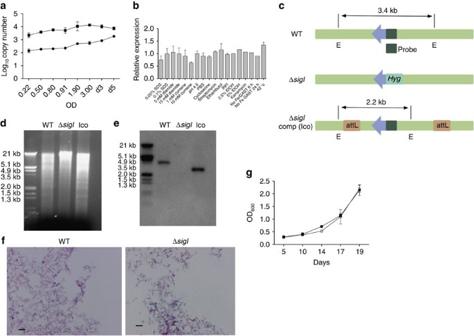Figure 1:sigIexpression and validation ofM.tb.ΔsigI. (a) Transcript copy numbers ofsigI(closed circle) andsigA(closed square) duringM.tb.growth in culture. (b) Using copy number,sigItranscription was analysed under stress conditions (relative to no stress conditions). The following stress conditions were analysed: detergent (SDS), disulphide (diamide), oxidative (cumene), acid (pH 4.5), antibiotic (cycloserine, streptomycin, ethambutol, INH and kanamycin), ethanol (EtOH), low iron (no Fe GAST) and heat shock (42 °C). (c) Diagram of the restriction map for Southern blotting of wild-type, ΔsigIand thesigI-complemented (Ico)M.tb.strains. Arrow indicatessigIgene. E:EcoRIrestriction site.Hyg: hygromycin resistance gene. (d) Agarose gel ofEcoRI-digested genomic DNA for Southern blotting. (e) Southern blot with probe (primers described inSupplementary Table S2). (f) Acid-fast staining of wild-type and ΔsigImutantM.tb.strains. Scale bar: 5 μm. (g) Growth curves for wild-type (open circle) and ΔsigI(closed square)M.tb.strains. Three biological replicates of all experiments were performed, and error bars represent s.d. Figure 1: sigI expression and validation of M.tb. Δ sigI . ( a ) Transcript copy numbers of sigI (closed circle) and sigA (closed square) during M.tb. growth in culture. ( b ) Using copy number, sigI transcription was analysed under stress conditions (relative to no stress conditions). The following stress conditions were analysed: detergent (SDS), disulphide (diamide), oxidative (cumene), acid (pH 4.5), antibiotic (cycloserine, streptomycin, ethambutol, INH and kanamycin), ethanol (EtOH), low iron (no Fe GAST) and heat shock (42 °C). ( c ) Diagram of the restriction map for Southern blotting of wild-type, Δ sigI and the sigI -complemented (Ico) M.tb. strains. Arrow indicates sigI gene. E: EcoRI restriction site. Hyg : hygromycin resistance gene. ( d ) Agarose gel of EcoRI -digested genomic DNA for Southern blotting. ( e ) Southern blot with probe (primers described in Supplementary Table S2 ). ( f ) Acid-fast staining of wild-type and Δ sigI mutant M.tb. strains. Scale bar: 5 μm. ( g ) Growth curves for wild-type (open circle) and Δ sigI (closed square) M.tb. strains. Three biological replicates of all experiments were performed, and error bars represent s.d. Full size image To examine the role of sigI more closely, we constructed a sigI deletion mutant and the corresponding complemented strain ( Fig. 1c ), both of which were confirmed by Southern blot ( Fig. 1d,e ). The sigI mutant displayed normal cellular morphology as observed by acid-fast staining ( Fig. 1f ) and growth rate in liquid culture ( Fig. 1g ). To identify the SigI regulatory network, we compared global gene expression patterns between the Δ sigI mutant and the parent wild-type strain using microarray ( Supplementary Table S1 ). As the microarray analyses served as a screening tool for the identification of SigI-regulated genes, the complemented strain was not included in the microarray studies. The SigI regulon identified included an ATP synthase ( Rv1304 ), heat shock proteins ( Rv0440 , Rv0350 and Rv3417 ) and katG . These data supported the role for SigI during heat shock ( Fig. 2a ). In addition to its ability to activate INH, the KatG catalase-peroxidase has been reported to have a detoxification role during oxidative stress, and has been found to be essential for full virulence in macrophage and mouse infection models [14] , [15] , [16] , [17] . This manuscript describes the follow-up validation and further characterization of the relationship between sigI and katG as suggested in our microarray screen. 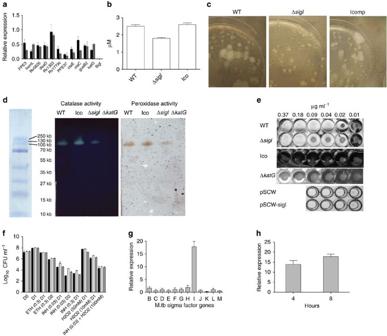Figure 2:In vitrocharacterization ofM.tb.ΔsigI. (a) The downregulation of genes, includingkatG, which were identified by microarray in the ΔsigImutant, was confirmed by qRT–PCR. Data represent gene expression (based on copy number) of the mutant compared with wild-type. Black bars represent bacteria at OD1, and dark grey bars represent bacteria at OD2. (b) Catalase activity within total cell lysates from wild-typeM.tb., the ΔsigImutant and the complemented strain (Icomp). (c) Catalase activity from bacteria growing on a 7H10 agar plate was detected with 10% H2O2. (d) Bacterial lysates were resolved by native PAGE. Catalase activity was visualized using 1% ferric chloride and 1% potassium ferricyanide. Peroxidase activity was visualized using a solution of 0.5 mg ml−1p-diaminobenzidine and 3 mM H2O2. (e) INH MIC assay results for wild-type, Δsig, and complemented (Ico)M.tb.strains, as well as thesigIoverexpressing strain (pSCW-sigI) and its empty vector control strain (pSCW). (f) Wild-type (black bars), ΔsigImutant (light grey bars) and complement (dark grey bars) strains were exposed to INH, ETH, H2O2and INH+H2O2for 1 or 2 days, and then plated on 7H10 agar for CFU enumeration. The combined INH and H2O2exposure was for 1 day. The ETH and INH concentrations are in μg ml−1, and the H2O2concentration is in mM. (g) Expression levels ofM.tb. sigB-sigMfollowing 4 h of acetamide-induced overexpression ofsigI(relative to expression before acetamide exposure). (h)M.tb. sigIexpression after 4 and 8 h of acetamide-induced expression. Three biological replicates of all experiments were performed, and error bars represent s.d. Figure 2: In vitro characterization of M.tb. Δ sigI . ( a ) The downregulation of genes, including katG , which were identified by microarray in the Δ sigI mutant, was confirmed by qRT–PCR. Data represent gene expression (based on copy number) of the mutant compared with wild-type. Black bars represent bacteria at OD1, and dark grey bars represent bacteria at OD2. ( b ) Catalase activity within total cell lysates from wild-type M.tb. , the Δ sigI mutant and the complemented strain (Icomp). ( c ) Catalase activity from bacteria growing on a 7H10 agar plate was detected with 10% H 2 O 2 . ( d ) Bacterial lysates were resolved by native PAGE. Catalase activity was visualized using 1% ferric chloride and 1% potassium ferricyanide. Peroxidase activity was visualized using a solution of 0.5 mg ml −1 p -diaminobenzidine and 3 mM H 2 O 2 . ( e ) INH MIC assay results for wild-type, Δ sig , and complemented (Ico) M.tb. strains, as well as the sigI overexpressing strain (pSCW-sigI) and its empty vector control strain (pSCW). ( f ) Wild-type (black bars), Δ sigI mutant (light grey bars) and complement (dark grey bars) strains were exposed to INH, ETH, H 2 O 2 and INH+H 2 O 2 for 1 or 2 days, and then plated on 7H10 agar for CFU enumeration. The combined INH and H 2 O 2 exposure was for 1 day. The ETH and INH concentrations are in μg ml −1 , and the H 2 O 2 concentration is in mM. ( g ) Expression levels of M.tb. sigB - sigM following 4 h of acetamide-induced overexpression of sigI (relative to expression before acetamide exposure). ( h ) M.tb. sigI expression after 4 and 8 h of acetamide-induced expression. Three biological replicates of all experiments were performed, and error bars represent s.d. Full size image Catalase production is decreased in the M.tb . Δ sigI mutant To determine whether the association between sigI deficiency and decreased katG expression was functionally significant, we examined the catalase-peroxidase activity of the Δ sigI mutant upon exposure to hydrogen peroxide. As shown in Fig. 2b,c , this activity was decreased in the mutant compared with wild-type bacteria, as well as in the bacterial lysates ( Fig. 2d ). The Δ katG mutant was devoid of detectable catalase activity ( Fig. 2d ), as has been well documented [17] . These data indicated that SigI has a role in the regulation of katG expression, but that other transcriptional mechanisms maintain a baseline level of katG expression. The M.tb. Δ sigI mutant exhibits resistance to INH In view of the fact that KatG is necessary for the activation of INH [12] , we investigated whether SigI-mediated expression of katG affected the organism's resistance to this antibiotic. We first determined the minimal inhibitory concentration–90% (MIC 90 ) of INH for the Δ sigI mutant, wild-type and complemented strains, and the well-characterized INH-resistant mutant Δ katG [17] . The Δ katG mutant lacks catalase-peroxidase activity altogether and is highly resistant to INH with an MIC 90 of 10 μg ml −1 (ref. 12 ) ( Fig. 2e ). As shown in Fig. 2e , the MIC 90 of the Δ sigI mutant was 0.18 μg ml −1 , four times higher than the wild-type strain (MIC 90 =0.04 μg ml −1 ), while the complement strain exhibited similar INH susceptibility as wild-type M.tb . As ethionamide (ETH) is an anti-TB drug that inhibits the product of inhA without a need for KatG-dependent activation [8] , we also tested the susceptibility of the Δ sigI mutant and related strains to ETH in order to evaluate if the Δ sigI mutant's INH resistance was mediated by katG - or inhA -dependent pathways. Bacteria were treated with INH, ETH and H 2 O 2 at various concentrations, and bacterial survival was determined after 24 and 48 h. We observed no difference in survival of ETH-treated bacteria compared with wild-type, whereas the Δ sigI mutant exhibited higher survival when exposed to INH ( Fig. 2f ). These data indicate that the M.tb. Δ sigI mutant's resistance to INH is due to reduced SigI-dependent katG expression, rather than from inhA -related gene regulation. An interesting additional finding was the observation that the Δ sigI mutant expressed sufficient catalase/peroxidase activity to protect from H 2 O 2 stress to near wild-type levels ( Fig. 2d,f ). The wild-type and Δ sigI bacteria had similar survival when exposed to H 2 O 2 and INH simultaneously, again indicating equivalent responses to H 2 O 2 . This may be due to a mechanism where the Δ sigI mutant expresses sufficient catalase/peroxidase activity to protect from H 2 O 2 oxidative damage despite compromised ability to activate INH. Overexpression of sigI results in increased susceptibility to INH To differentiate whether SigI directly regulates katG transcription or if katG expression is regulated by other SigI-dependent cofactors, we constructed a conditionally overexpressing sigI merodiploid strain in which the second copy of sigI was expressed from the acetamide-inducible promoter P ace ( Fig. 2g,h ). We also measured the MIC to INH for the sigI overexpression strain, and this strain exhibited a lower MIC (0.02 μg ml −1 ) than either the wild-type or control strain carrying the empty vector ( Fig. 2e ). These data further indicate a specific role for SigI in the bacterial response to INH. SigI directs transcription of katG Transcription of M.tb . katG has been shown to occur from two different promoters: one upstream of the furA gene, which itself is upstream of katG , and also one directly upstream of katG , between furA and kat G [18] . We utilized an in vitro transcription (IVT) assay to test directly whether SigI could direct transcription of katG from either of these promoter sequences. We expressed and purified recombinant SigI protein to >98% purity for use in the assembly of an RNA polymerase holoenzyme; purified recombinant SigI was combined with the Escherichia coli RNA core polymerase (that is, RNA polymerase lacking a sigma factor component). This SigI-containing enzyme complex was then incubated in a reaction buffer containing a DNA template comprising the katG gene, including the promoter sequence 379-bp upstream. Any transcripts generated by the IVT reaction were then amplified and evaluated by RT–PCR. Although the SigI-containing RNA polymerase holoenzyme was unable to direct transcription from the non-SigI-regulated gene Rv1186 , SigI-directed transcription was detected from the katG promoter, providing direct evidence that SigI can direct transcription from the katG promoter located 379-bp upstream of the gene ( Fig. 3a ). 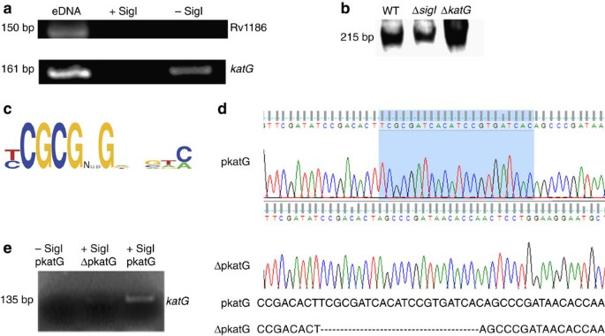Figure 3: SigI transcribes thekatGgene. (a) SigI-containing RNA polymerase holoenzyme was able to direct transcription from the promoter region 379-bp upstream of thekatGgene. After transcription by SigI, the gene product was amplified by RT–PCR. The open reading frame regionRv1186was used as a negative control for IVT, as SigI does not direct transcription of this gene. (b) Total bacterial lysates from wild-type and ΔsigIstrains were utilized as RNA polymerase component in an IVT assay in which the promoter region 33-bp upstream ofkatGwas used as the DNA template. (c) Putative SigI-binding motif as identified from upstream sequences of the genes identified by microarray to be a part of the SigI regulon. (d) Nucleotide sequence of thekatGpromoter; the shaded region indicates the deletion. (e) SigI cannot direct transcription from an IVT template in which the putative SigI-binding motif has been deleted (from promoter region 33-bp upstream ofkatG, ΔpkatG). Three biological replicates of all experiments were performed. Figure 3: SigI transcribes the katG gene. ( a ) SigI-containing RNA polymerase holoenzyme was able to direct transcription from the promoter region 379-bp upstream of the katG gene. After transcription by SigI, the gene product was amplified by RT–PCR. The open reading frame region Rv1186 was used as a negative control for IVT, as SigI does not direct transcription of this gene. ( b ) Total bacterial lysates from wild-type and Δ sigI strains were utilized as RNA polymerase component in an IVT assay in which the promoter region 33-bp upstream of katG was used as the DNA template. ( c ) Putative SigI-binding motif as identified from upstream sequences of the genes identified by microarray to be a part of the SigI regulon. ( d ) Nucleotide sequence of the katG promoter; the shaded region indicates the deletion. ( e ) SigI cannot direct transcription from an IVT template in which the putative SigI-binding motif has been deleted (from promoter region 33-bp upstream of katG , ΔpkatG). Three biological replicates of all experiments were performed. Full size image Next, we evaluated the transcriptional activities present in the cytoplasm of the Δ sigI mutant compared with wild-type. Bacterial lysates prepared from wild-type M.tb. , the Δ sigI mutant, as well as the Δ katG mutant, were used for IVT experiments using a katG template with the promoter located 33-bp upstream of the gene. As presented in Fig. 3b , lysates from the Δ sigI mutant were associated with significantly decreased katG transcription, further demonstrating a direct SigI transcriptional effect in the expression of katG . These transcription-based assays thus indicate that SigI transcribes katG from both of its known promoters [18] . Based on this information and the upstream sequences of the genes comprising the putative SigI regulon ( Fig. 2a ), we identified a possible SigI-binding motif ( Fig. 3c ). To validate this putative SigI-binding motif, we next performed an IVT assay using a katG template with this motif deleted from the promoter sequence immediately upstream of the katG gene ( Fig. 3d ). Removal of this short sequence nearly abolished the ability of SigI to direct transcription of katG ( Fig. 3e ), thus confirming SigI-mediated transcription of katG . Taken together with our results, these findings indicate a possible role for SigI-mediated katG expression in the context of INH treatment. M.tb. Δ sigI is not attenuated in cell culture infections M.tb. strains lacking a functional KatG enzyme are severely attenuated in virulence in both macrophage and mouse infection models [15] , [17] , suggesting that a decrease in the SigI-dependent expression of katG could be associated with defective growth and virulence in these model systems. Therefore, we analysed the ability of the Δ sigI mutant to survive within J774A.1 murine macrophages. Activated cells were infected with wild-type M.tb. or the Δ sigI or Δ katG mutants, and intracellular bacterial loads were determined after 24 h, 3 days and 6 days post infection. As shown in Fig. 4a , survival of the Δ sigI strain was similar to wild-type, while the Δ katG mutant was attenuated in growth, indicating that the Δ sigI mutant was not associated with a decrease in virulence. Furthermore, when J774A.1 cells were co-infected with both wild-type and Δ sigI M.tb. , the strains grew equally well and with the same growth kinetics as in singly infected cells, again indicating that the Δ sigI strain was not attenuated for growth in murine macrophage-like cells ( Fig. 4b ). 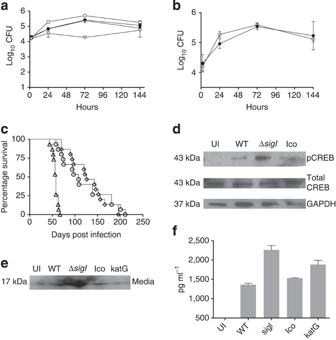Figure 4:M. tb. ΔsigImutant strain is not attenuated in cells or mice. (a) J774A.1 murine macrophages were infected with wild-typeM.tb.(closed circle), the ΔsigImutant (open circle), the complemented strain (closed triangle) and the ΔkatGmutant (open triangle). (b) J774A.1 cells were co-infected with wild-typeM.tb.(closed circle) and the ΔsigImutant (open circle). (c) Time-to-death for three groups each of 20 Balb/c mice that were infected with an inoculum that implanted∼3.7 log10bacteria per lung by aerosol; wild-type (open circle), ΔsigI(open triangle) and complement strain (open diamond). (d) CREB phosphorylation was measured by western blot inM.tb.-infected J774A.1 cells at 12 h. (e) TNF-α production was measured in infected J774A.1 by western blot. (f) TNF-α production was measured in infected J774A.1 by ELISA. The time-to-death experiment was performed once. Three biological replicates of all other experiments were performed, and error bars represent s.d. Figure 4: M . tb . Δ sigI mutant strain is not attenuated in cells or mice. ( a ) J774A.1 murine macrophages were infected with wild-type M.tb. (closed circle), the Δ sigI mutant (open circle), the complemented strain (closed triangle) and the Δ katG mutant (open triangle). ( b ) J774A.1 cells were co-infected with wild-type M.tb. (closed circle) and the Δ sigI mutant (open circle). ( c ) Time-to-death for three groups each of 20 Balb/c mice that were infected with an inoculum that implanted ∼ 3.7 log 10 bacteria per lung by aerosol; wild-type (open circle), Δ sigI (open triangle) and complement strain (open diamond). ( d ) CREB phosphorylation was measured by western blot in M.tb. -infected J774A.1 cells at 12 h. ( e ) TNF-α production was measured in infected J774A.1 by western blot. ( f ) TNF-α production was measured in infected J774A.1 by ELISA. The time-to-death experiment was performed once. Three biological replicates of all other experiments were performed, and error bars represent s.d. Full size image M.tb. Δ sigI is hypervirulent in BALB/c mice We next evaluated whether this trend would extend to in vivo infections. Groups of 20 female BALB/c mice were infected by the aerosol route with wild-type M.tb. , the Δ sigI mutant, or the complemented Δ sigI strain and monitored for time-to-death; day 1 colony-forming unit (CFU) counts for each strain were 3.75, 3.86 and 3.75 log 10 CFU, respectively. Interestingly, compared with the wild-type and complemented strains, infection with the Δ sigI mutant was associated with more rapid death of the mice, with half of the Δ sigI -infected mice dying by day 58 post infection, while the corresponding value for wild-type and complement strain-infected mice was day 139 and day 146, respectively ( Fig. 4c ). Thus, the M.tb. Δ sigI mutant strain displayed a hypervirulent phenotype in this time-to-death mouse infection model. As the in vivo data were contrary to our hypothesis that the Δ sigI mutant would exhibit attenuated growth and virulence in our model systems, we examined an additional parameter associated with M.tb. virulence, namely CREB phosphorylation and tumour necrosis factor (TNF)-α production. Recent reports from our laboratory and others have indicated that upon infection, an initial increase in TNF-α levels benefit these organisms, and that virulent mycobacteria actively modulate host signalling to increase the expression of this pro-inflammatory cytokine [19] , [20] , [21] . The Δ sigI mutant, in contrast to the wild-type or complemented strains, induced increased CREB phosphorylation within infected J774A.1 cells ( Fig. 4d ), as well as increased TNF-α secretion ( Fig. 4e,f ). These data are in agreement with the in vivo results, indicating that the Δ sigI mutant is not attenuated for growth or virulence within these model systems, despite exhibiting KatG-associated INH resistance. The infection with the Δ katG mutant may have also induced increased TNF-α secretion from these cells, as we observed an increase in TNF-α in the culture supernatant as measured by enzyme-linked immunosorbent assay (ELISA) ( Fig. 4f ) that was not observed in western blot analysis ( Fig. 4e ). Thus, from our data, the role of TNF-α is unclear in its relationship to the attenuated Δ katG mutant. Lack of sigI confers low-level resistance to INH in vivo To address the relevance of sigI deletion in M.tb. resistance to INH, we infected female BALB/c mice with wild-type or Δ sigI M.tb. (with day 1 log 10 CFU counts of 3.44 and 3.71, respectively), and treatment with INH was initiated at 14 days post infection. For each strain, INH was administered by oral gavage at 0.5, 1.5 and 6.0 mg kg −1 per day, and lung CFU counts were obtained at 28 and 56 days post infection (that is, after 14 and 42 days, respectively, of INH treatment). All Δ sigI -infected mice that did not receive INH or were treated at the lowest dose (0.5 mg kg −1 per day) died before the end of the experiment ( Fig. 5a ), again indicating increased virulence of this strain compared with wild-type, even in the presence of low-level INH. In addition, Δ sigI -infected mice receiving either 1.5 or 6.0 mg kg −1 per day of INH had significantly higher lung CFU counts at both day 28 and day 56 post infection compared with mice infected with wild-type M.tb. ( Fig. 5b ). We hypothesize that the increased survival of the Δ sigI strain is related to the low-level INH resistance displayed by this strain in vitro ; however, it is possible that this observation is due to the increased virulence of the strain. Taken together, these data confirm the virulent phenotype of the Δ sigI mutant strain and demonstrate that lack of SigI function is associated with increased survival in the presence of INH. 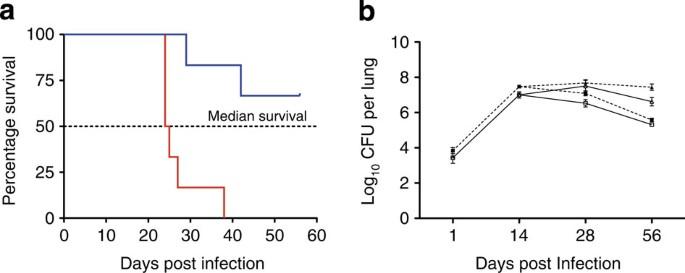Figure 5: The ΔsigImutant strain is resistant to INHin vivo. Two groups of 50 BALB/c mice each were infected with wild-type and ΔsigI M.tb.with an inoculum that implanted∼3.5 log10bacteria per lung by aerosol. Fourteen days post infection, INH was administered to the mice daily (5 days per week) by oral gavage at doses of 0.5, 1.5 and 6.0 mg kg−1per day. (a) Time-to-death analysis of infected mice treated with 0.5 mg kg−1INH per day. Blue line: wild-typeM.tb.; red line: ΔsigImutant. (b) CFU counts in mouse lungs for mice treated or untreated with INH at 1.5 and 6.0 mg kg−1per day. All untreated mice infected with the ΔsigIstrain died before the day 56 time point. Triangle: sham treatment (no INH). Square: 1.5 mg kg−1per day INH. Circle: 6.0 mg kg−1per day INH. Solid lines: wild-type. Dashed lines: ΔsigI. This experiment was performed once, with five mice per treatment group. Error bars represent s.d. Figure 5: The Δ sigI mutant strain is resistant to INH in vivo . Two groups of 50 BALB/c mice each were infected with wild-type and Δ sigI M.tb. with an inoculum that implanted ∼ 3.5 log 10 bacteria per lung by aerosol. Fourteen days post infection, INH was administered to the mice daily (5 days per week) by oral gavage at doses of 0.5, 1.5 and 6.0 mg kg −1 per day. ( a ) Time-to-death analysis of infected mice treated with 0.5 mg kg −1 INH per day. Blue line: wild-type M.tb. ; red line: Δ sigI mutant. ( b ) CFU counts in mouse lungs for mice treated or untreated with INH at 1.5 and 6.0 mg kg −1 per day. All untreated mice infected with the Δ sigI strain died before the day 56 time point. Triangle: sham treatment (no INH). Square: 1.5 mg kg −1 per day INH. Circle: 6.0 mg kg −1 per day INH. Solid lines: wild-type. Dashed lines: Δ sigI . This experiment was performed once, with five mice per treatment group. Error bars represent s.d. Full size image Mathematical models have indicated that the relative fitness of drug-resistant M.tb. strains is the most important determinant when predicting the spread and epidemic potential of MDR- and XDR-TB [2] , [22] . Here, we have presented a possible mechanism of INH resistance, that is, loss of sigI and the associated SigI-dependent katG expression. The Δ sigI mutant did not exhibit diminished growth or virulence within mouse infection models, and in fact our data demonstrate that this mutant strain was more virulent than wild-type M.tb. under the conditions tested. Furthermore, we have shown that the loss of sigI results in increased bacterial survival in the presence of INH, indicating an in vivo role for SigI in INH resistance. These findings could have significant implications for the spread of drug-resistant M.tb. strains. Recently, Ando et al . [23] have characterized INH-resistant human clinical isolates of M.tb. in Japan. In their analysis of 108 INH-resistant isolates, they identified three unique mutations in the intergenic region upstream of katG in 4% of the isolates. Three of these isolates did not contain additional mutations in the examined sequences ( katG, inhA promoter , aphC, ndh or kasA-kasB ), while one isolate also contained a mutation in the inhA promoter region. These recent findings indicate that changes in the katG promoter sequence can affect resistance to INH, and that this mode of INH resistance is relevant in human TB. While the putative SigI-binding site that we identified was not mutated in these INH-resistant strains, this work by Ando et al . indicates that alterations in the katG promoter region influence susceptibility to INH. Thus, these findings support our hypothesis that SigI-mediated transcription of katG may be associated with M.tb. susceptibility to INH. Although M.tb. lacking KatG function exhibit attenuated fitness for growth compared with wild-type M.tb. , a second compensatory mutation has been identified, which results in a regain of fitness, namely mutations in the ahp gene, which encodes a peroxidase [12] . Therefore, the generation of INH resistance through this mechanism can be thought of as a two-step process whereby the initial katG mutation is associated with a fitness loss, followed by a secondary, compensatory mutation in ahp , which may increase the ability of the drug-resistant strain to survive in the community. In this communication, we have described an alternative pathway towards INH resistance in which a step towards drug (or multidrug) resistance, that is, mutation of sigI , is not associated with a fitness cost. Construction of mutant strains The Δ sigI mutant was created using a suicide vector approach using the plasmid pCK0686 (ref. 24 ). The upstream-flanking region of the sigI gene was amplified by PCR using primers sigIP1 and sigIP2 ( Supplementary Table S2 ) and directionally cloned into pCK0686 using Nde I and Spe I restriction sites. Similarly, the downstream-flanking region of the sigI gene was amplified by PCR using primers sigIP3 and sigIP4 and then directionally cloned into pCK0686 using PacI and XhoI restriction sites to create pKOsigI. The suicide vector pKOsigI was then transformed into electrocompetent M.tb. using a Bio-Rad E. coli Pulser, and transformants were selected using 7H10 plates containing Hygromycin B (50 μg ml −1 ). Double crossover events leading to a proper gene disruption were isolated by selection on plates containing Hygromycin B (50 μg ml −1 ) and 5% sucrose. A complemented strain was constructed using the integrating plasmid pMH94. A 4.1-kb region containing the sigI gene was amplified by PCR using primers psigIcomp5 and psigIcomp6 ( Supplementary Table S2 ), and the resulting amplicon was cloned into pMH94 using the XbaI restriction site. The resulting complementation plasmid was transformed into electrocompetent Δ sigI cells, and transformants were selected using both kanamycin (10 μg ml −1 ) and hygromycin B (50 μg ml −1 ). Purification of recombinant SigI Recombinant SigI was purified as carboxy terminal His-tagged recombinant protein. The entire open reading frame of the M.tb. sigI gene was PCR amplified using primers pETsigI1 and pETsigI2 ( Supplementary Table S2 ). The amplicon was digested with Nde I and Hin dIII, and ligated to Nde I and HindIII-digested pET22b (+) (Novagen). The resulting vector, pET-sigI, was then transformed into E. coli BL21(DE3) strain. SigI overexpression was induced using 1 mM isopropyl-β- D -thiogalactopyranoside, and after 3 h of induction, the cells were harvested and disrupted by sonication in binding buffer (50 mM Tris–Cl, 0.5 M NaCl, 10 mM imidazol and 8 M urea). The lysate was applied to a Histrap FF crude column (GE Healthcare) and purified using an FPLC system (Amersham). The purity of the protein was visualized using SDS–PAGE, and protein concentration was determined using the Bradford method. Conditionally overexpressing sigI Previously, we constructed sigF and sigB overexpression vectors pSCW35 and pSCW40 containing an acetamide promoter– sigF or sigB fusion gene, respectively, as well as a control vector pSCW38, containing only the acetamide promoter [25] . To overexpress sigI in M.tb. , the entire sigI gene was amplified by PCR using primers pACEI1 and pACEI2 and directionally cloned into pSCW35 using NdeI and PacI restriction sites. The resulting vector, pSCW-sigI, was transformed into electrocompetent M.tb. and transformants were isolated on 7H10 plates containing kanamycin (10 μg ml −1 ). Microarray Total RNA was extracted from wild-type M.tb. and Δ sigI mutant at both OD 600 =1 and OD 600 =2. One microgram of RNA was reverse-transcribed with random hexamers (Invitrogen), and the resulting complementary DNA was labelled with Cy3-dCTP or Cy5-dCTP, and competitively hybridized to whole-genome arrays. Arrays were scanned using an Axon 4000B scanner and images were analysed using GenePix pro 4.0 software. The resulting data were normalized to the total integrated intensity across both channels, and the ratio of Cy5 and Cy3 was compared and calculated. Q value was obtained using SAM (Significance Analysis of Microarrays). The microarray data discussed in this publication have been deposited in NCBI's Gene Expression Omnibus [26] and are accessible through GEO series accession number GSE35231. Real-time RT–PCR The Δ sigI mutant was confirmed by real-time RT–PCR from RNA isolated from M.tb. CDC1551. Bacterial cells were centrifuged, washed with PBS and resuspended in Trizol reagent (Invitrogen) followed by bead beating with 0.1 mm diameter silica beads at 5000 r.p.m. After centrifugation at 10,000× g for 5 min at 4 °C, the supernatants were collected, treated with chloroform and centrifuged again to collect the aqueous phase. Finally, RNA was precipitated with one volume of isopropyl alcohol, washed with 75% ethanol and dried. About 1 μg of DNase I-treated RNA was transcribed with Superscript II Reverse Transcriptase (Invitrogen) using random primers (Invitrogen). Real-time PCR was carried out using IQ SYBR Green I PCR kit (Bio-Rad). The cDNA and RT primer set ( Supplementary Table S2 ) were added to each reaction and specific amplification was detected at the extension cycle. The threshold cycle ( C T ) was converted to copy numbers using a DNA standard curve. In vitro transcription assay The DNA templates including the putative katG promoter regions were prepared by PCR using primers katG1 and katG2 ( Supplementary Table S2 ). Two picomoles of E. coli RNA core polymerase (Epicentre) were incubated with 20 pmol of purified sigma factor protein for 30 min in transcription assay buffer (10 mM Tris, 50 mM KCl, 10 mM MgCl 2 , 0.1 mM EDTA and 0.25 μg μl −1 bovine serum albumin), then 0.09 μg of template DNA was added and incubated with 0.35-mM 11-biotin UTP, 1 mM ATP, 1 mM CTP, 1 mM GTP and 0.65 mM UTP mixture [25] . The template with the putative SigI-binding motif deleted was generated using the mega-primer method [27] . Survival of sigI mutant with several antibiotics and determination of the MIC Survival of Δ sigI mutant with INH, ETH and H 2 O 2 was analysed by the addition of INH (0.03 and 0.3 μg ml −1 ), ETH (0.3 μg ml −1 ) and H 2 O 2 (50 and 100 mM) to cultures for 24 and 48 h; aliquots were plated onto 7H10 agar. The MIC of INH for sigI mutant was also checked using 24–0.01 μg ml −1 INH. INH was added to the media and the growth of wild-type, Δ sigI mutant, the sigI- complemented strain and the katG deletion mutant strain were checked after 7 and 14 days. Catalase activity assay Whole-cell lysates from wild-type and the Δ sigI deletion mutant were prepared using a bead beater method. Ten micrograms of total protein was used to measure the catalase activity using a catalase assay kit (Calbiochem). Catalase and peroxidase activity were also measured using a gel staining method where the cell lysate was separated using a 10% non-denaturing PAGE gel. After electrophoresis, the gel was incubated in 0.03% H 2 O 2 for 5 min and washed. Catalase activity was visualized by soaking the gel in a solution containing 1% (w/v) ferric chloride and 1% (w/v) potassium ferricyanide. Peroxidase activity was detected by incubating in detection solution (0.5 mg ml −1 p -diaminobenzidine and 3 mM H 2 O 2 ). Macrophage infection J774A.1 cells were cultivated in cRPMI (2 mM glutamine and 10% FBS) and activated by incubating with interferon-γ (500 U ml −1 ) for 12 h, followed by incubation with lipopolysaccharide (200 ng ml −1 ) for 3 h before infection. After washing the macrophages three times with cRPMI, 10 5 bacteria were used to infect macrophage culture at an multiplicity of infection of 1:1. After 2 h of infection, macrophages were washed five times with RPMI media, and cultivated with cRPMI with 5% CO 2 at 37 °C. Macrophages were harvested, washed three times with RPMI and then lysed using 0.1% triton X-100 in PBS at each time point (2 h, 3 days and 6 days after infection). Macrophage lysate was plated on 7H10 plates for enumeration of bacterial CFU. TNF-α and CREB measurement TNF-α production was measured using the DuoSet mouse TNF-α ELISA kit (R&D Biosystems) and by western blot using anti-mouse TNF-α antibody with biotin conjugate (Invitrogen), diluted 1:1,000. CREB phosphorylation was measured by western blot using phospho-CREB antibody at 1:2,000, total CREB antibody at 1:3,000 (both from Cell Signaling) and GAPDH antibody at 1:35,000 (Sigma). Virulence assessment of Δ sigI mutant Three groups of 20 randomized six-week-old female BALB/c mice (Charles River) were infected with either wild-type, Δ sigI or the complemented strain using a Middlebrook inhalation exposure system (Glas-Col) with 10 ml of a diluted mid-log phase M.tb. culture intended to implant ∼ 1,000 bacilli in the lungs. One day post infection, three mice from each group were killed in order to determine the implanted dose. Mice were observed until death, with the time of each death recorded. Mice were maintained in isolator cages, with not more than five mice per cage, in the Johns Hopkins Center for Tuberculosis Research Animal Biosafety Level 3 facility. All animal experiments were carried out in strict accordance with the recommendations in the Guide for the Care and Use of Laboratory Animals of the National Institutes of Health, and all procedures were approved by the Johns Hopkins University Animal Care and Use Committee. Bacterial survival in vivo during INH treatment Two groups (50 mice per group) of randomized 6-week-old female BALB/c mice (Charles River) were infected by aerosol as described above with either wild-type or ΔsigI M.tb. with implants of ∼ 3.5 log 10 bacilli into the lung. Five mice from each group were killed on day 1 to determine implant dose, and an additional five mice from each group were killed on day 14 to determine lung bacterial burden before initiating treatment. Starting on day 14 post infection, the remaining mice were given INH five days per week via oral gavage (200 μl total volume) at either 0, 0.5, 1.5 or 6.0 mg kg −1 per day (INH was dissolved in water). Four mice from each group were killed at day 28, and all remaining mice were killed at day 56 post infection. Lung homogenates were plated on selective 7H11 agar plates for CFU determination, and on days 28 and 56, lung homogenates were also plated on selective 7H11 agar plates containing 0.1 μg ml −1 . Accession codes: The microarray data have been deposited in the Gene Expression Omnibus under accession number GSE35231 . How to cite this article: Lee, J-H. et al . Isoniazid resistance without a loss of fitness in Mycobacterium tuberculosis . Nat. Commun. 3:753 doi: 10.1038/ncomms1724 (2012).